Loss of polarity protein AF6 promotes pancreatic cancer metastasis by inducing Snail expression Pancreatic cancer (PC) is a particularly lethal form of cancer with high potential for metastasis to distant organs. Disruption of cell polarity is a hallmark of advanced epithelial tumours. Here we show that the polarity protein AF6 (afadin and MLLT4) is expressed at low levels in PC. We demonstrate that depletion of AF6 markedly promotes proliferation and metastasis of PC cells through upregulation of the expression of Snail protein, and this requires the nuclear localization of AF6. Furthermore, AF6 deficiency in PC cells leads to increased formation of a Dishevelled 2 (Dvl2)–FOXE1 complex on the promoter region of Snail gene, and activation of Snail expression. Altogether, our data established AF6 as a potential inhibitor of metastasis in PC cells. Targeting the Dvl2–FOXE1–Snail signalling axis may thus represent a promising therapeutic strategy. Pancreatic cancer (PC) is a major leading cause of cancer-related mortality worldwide. In the US alone, ∼ 46,420 new cases and ∼ 39,590 deaths are predicted for 2014 (ref. 1 ). Currently, diagnosis of PC is only possible for those in advanced state and the prognosis of PC remains the worst in any major malignancy. For example, in cases of pancreatic ductal adenocarcinoma (PDAC), a particularly lethal form of PC, the median survival of all patients is still <6 months, and the 5-year relative survival rate after diagnosis is <6%. Early invasion and metastasis have so far been well accepted as the leading feature and main cause of death in PC. However, mechanistic understanding of the highly metastatic potential of PC remains incomplete and novel biomarkers or targets are yet to be identified for diagnosing or treating PC. Meanwhile, disruption of cell polarity and tissue disorganization is a hallmark of advanced epithelial tumours [2] . AF6 (also known as afadin and MLLT4) is well known as a key molecule essential for structural organization of cell–cell junctions and development. The human AF6 gene is located on chromosome 6 band q27 (ref. 3 ), and was originally identified as a fusion partner of the ALL-1 gene involved in acute lymphoblastic leukaemia [4] . AF6 is a multi-domain protein, consisting (from the N to C terminus) of two Ras-associating domains, a forkhead-associated domain, a dilute domain, a PDZ (PSD95/Dlg1/ZO-1) domain and three proline-rich regions (Pro) [5] , [6] , [7] . In rodents and humans, AF6 is expressed in almost all epithelial tissues [8] mainly with two isoforms: a long isoform containing the F-actin-binding domain (FA) and a short isoform lacking the FA domain; these versions are referred to as l- and s-afadin, respectively. Known interacting partners for AF6 include cytoskeletal components and those involved in cell adhesion [9] . AF6 knockout mice exhibit embryonic lethality with developmental defects at stages during and after gastrulation. The phenotypic changes observed with these mice include disorganization of the ectoderm, impaired migration of the mesoderm and loss of somites or other structures derived from both the ectoderm and the mesoderm [10] , [11] . Recently, expression of the AF6 gene was found to be aberrant in multiple cancer types, including leukaemia, ovarian and breast cancers [3] , [4] , [12] , [13] , [14] , [15] , [16] , but the specific roles that AF6 might play in tumorigenesis remain unclear. In this study, we employ three-dimensional (3D) cell culture systems, in vivo PC animal models and clinical samples to address the effect of AF6 loss on proliferation and metastasis of PC cells. We show that AF6 deficiency affects the Dishevelled 2 (Dvl2)-regulated recruitment of FOXE1 to the Snail promoter, resulting in activation of Snail gene transcription. Our findings demonstrate a role for AF6 in the regulation of invasion and metastasis AF6 is expressed at low levels in human PC As noted above, AF6 is produced in two functional isoforms (l- and s-afadin). To study the expression pattern of AF6 in PC, we first characterized the protein levels of AF6 isoforms in our pancreatic cell lines by using two different antibodies: an anti-AF6 antibody (Abcam) directed against l-afadin and an anti-AF6 antibody (BD) that recognizes both isoforms ( Fig. 1a ). Both antibodies detected a major band at 220 kDa in the immortalized human pancreatic ductal epithelial cell line (HPDE) and in another nine human PC cell lines, as well as in l-afadin-overexpressing Capan-1 cells. However, this band could not be detected by anti-AF6 antibody in s-afadin-overexpressing Capan-1 cells, indicating that the long isoform of AF6 (l-afadin) is expressed predominantly in these PC cells. 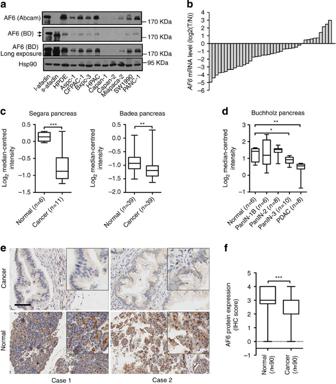Figure 1: AF6 is expressed at low levels in human pancreatic cancer. (a) Western blots of protein extracts derived from immortalized human pancreatic ductal epithelial cell line HPDE and nine other human pancreatic cancer cell lines; l-afadin- or s-afadin-overexpressing Capan-1 cells were used as positive controls. The anti-AF6 antibody recognizes an epitope corresponding to the last C-terminal amino-acid residues of l-afadin. The anti-AF6 antibody recognizes an epitope corresponding to the PDZ domain, which is present in both l-afadin and s-afadin. Up and down blank arrows indicate l-afadin or s-afadin, respectively. (b) Real-time PCR analysis of the mRNA expression ofAF6in 40 paired human pancreatic cancer tissues (T) and adjacent normal tissues (N). Data represent the mean±s.d. (n=3). (c) Box plots comparingAF6mRNA levels in normal pancreas and pancreatic cancer in published data sets from Oncomine. **P<0.01, ***P<0.001, Student’st-test. (d) The mRNA expression profiles ofAF6in normal pancreas, different stages of PanIN, and in PDAC. *P<0.05, **P<0.01, Student’st-test. (e,f) IHC staining for AF6 in adjacent normal and paired pancreatic cancer tissues (e). Box plots of AF6 protein expression assessed by blinded IHC analyses of 90 normal and paired pancreatic cancer tissues (f). ***P<0.001, Student’st-test. Scale bar, 100 μm. Figure 1: AF6 is expressed at low levels in human pancreatic cancer. ( a ) Western blots of protein extracts derived from immortalized human pancreatic ductal epithelial cell line HPDE and nine other human pancreatic cancer cell lines; l-afadin- or s-afadin-overexpressing Capan-1 cells were used as positive controls. The anti-AF6 antibody recognizes an epitope corresponding to the last C-terminal amino-acid residues of l-afadin. The anti-AF6 antibody recognizes an epitope corresponding to the PDZ domain, which is present in both l-afadin and s-afadin. Up and down blank arrows indicate l-afadin or s-afadin, respectively. ( b ) Real-time PCR analysis of the mRNA expression of AF6 in 40 paired human pancreatic cancer tissues (T) and adjacent normal tissues (N). Data represent the mean±s.d. ( n =3). ( c ) Box plots comparing AF6 mRNA levels in normal pancreas and pancreatic cancer in published data sets from Oncomine. ** P <0.01, *** P <0.001, Student’s t -test. ( d ) The mRNA expression profiles of AF6 in normal pancreas, different stages of PanIN, and in PDAC. * P <0.05, ** P <0.01, Student’s t -test. ( e , f ) IHC staining for AF6 in adjacent normal and paired pancreatic cancer tissues ( e ). Box plots of AF6 protein expression assessed by blinded IHC analyses of 90 normal and paired pancreatic cancer tissues ( f ). *** P <0.001, Student’s t -test. Scale bar, 100 μm. Full size image We next examined the expression pattern of AF6 in PC cells or clinical specimen. We found that the AF6 protein was expressed at low levels in most PC cell lines and highly expressed in the normal human pancreatic ductal epithelial cell line HPDE ( Fig. 1a ). In addition, real-time PCR revealed that AF6 messenger RNA (mRNA) was expressed at low levels (log 2 (T/N)≤−1) in 24 of 40 cancer samples and at higher levels in the paired normal tissues ( Fig. 1b ). These results were further confirmed by in silico analyses of two other independent data sets obtained from Oncomine [17] , [18] , [19] ( Fig. 1c ). In addition, in silico analyses showed that AF6 mRNA levels were expressed at low levels in PanIN-3 and PDAC compared with normal tissues in the context of the proposed multistep PDAC progression model [20] , [21] ( Fig. 1d ). Furthermore, immunohistochemical (IHC) staining of 90 paired normal and PC tissues revealed that AF6 protein levels were lower in PC specimens ( Fig. 1e,f ). Taken together, these results suggest that AF6 is expressed at lower levels in PC. Loss of AF6 promotes tumour proliferation and metastasis To characterize the effect of AF6 deficiency on the tumorigenicity of PC cells, we knocked down the expression of AF6 using virus-mediated RNA interference (RNAi; shAF6-1 and shAF6-2) in Bxpc-3 and HPAC cells ( Fig. 2b and Supplementary Fig. 1b ). We found that AF6 silencing induces gross changes in cell morphology in monolayer (2D) cell culture ( Fig. 2a and Supplementary Fig. 1a ). Previous work showed that 3D cell culture provides a powerful tool for investigating the molecular signals that specify epithelial tissue architecture [22] , [23] . We therefore extended our 2D analysis by using 3D cell culture. In contrast to control cells, AF6 -silenced cells formed larger spheroid-like structures and exhibited elevated invasive behaviour (as monitored by laminin V expression, a marker of basement membrane; Fig. 2a,c ; Supplementary Figs 1a,c and 2a ). Given that AF6 is a polarity protein, we further investigated the effect of AF6 deficiency on cell polarity in 3D culture. We first performed immunofluorescence analyses for E-cadherin, a protein responsible for maintaining baso-lateral cell adhesion and polarity. E-cadherin staining indicated that depletion of AF6 expression in Bxpc-3 cells disrupted the baso-lateral polarity ( Supplementary Fig. 2b ). As most human PC cell lines cannot form well polarized lumen structures in 3D culture, we used a non-tumorigenic human mammary epithelial cell-line (MCF-10A) model known to form 3D structures with well polarized out layers of cells by Day 8. To analyse changes in polarity, we monitored the orientation of the Golgi apparatus by staining (at Day 12) with the apical polarity marker GM130. In control cells cultured in 3D conditions, the Golgi always were oriented towards the apical side; in contrast, AF6-depleted MCF-10A cells cultured in 3D demonstrated a partial loss of the apical polarity of the Golgi, along with localization of GM130 to their baso-lateral surface ( Supplementary Fig. 2c ). Our results thus demonstrated that AF6 plays a role during the establishment of apical-basal axis of polarity. Diphenyltetrazolium bromide (MTT) proliferation and transwell invasion assays further indicated that depletion of AF6 expression in Bxpc-3 or HPAC cells significantly increased cellular proliferation and invasion ( Supplementary Fig. 3a,b ). Conversely, as shown in Supplementary Fig. 3c , cellular proliferation or invasion was significantly attenuated on overexpression of AF6 in Capan-1 or Capan-2 cells. These results suggested that loss of AF6 expression in PC cells promotes cell invasion and proliferation in vitro . 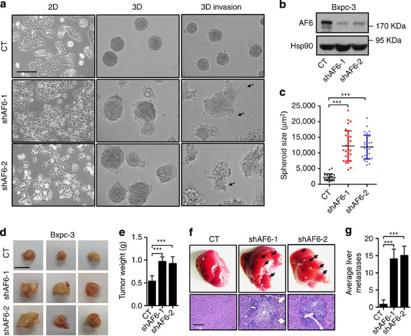Figure 2: Loss of AF6 promotes tumour proliferation and metastasis. (a) Phase-contrast images of Bxpc-3 cells stably expressing control (CT) or either of twoAF6shRNAs and grown as 2D, 3D or 3D invasion cultures (Day 10). Black arrows indicate invasive structures. Scale bar, 100 μm. (b) AF6 protein levels in Bxpc-3 cells harbouring control or either of twoAF6shRNAs. (c) The sizes of spheroids inawere measured. Data represent the mean±s.d. (n=30) from three separate experiments. ***P<0.001, Student’st-test. (d,e) Four-week-old nude mice were orthotopically transplanted with Bxpc-3 control (CT) or Bxpc-3 shAF6 cells (shAF6-1 and shAF6-2) (1 × 106cells per animal,n=7); tumours were harvested, photographed (d) and weighed at autopsy (Day 60). Results are presented as mean±s.d. (n=5) of calculated tumour weight (e). Scale bar, 1 cm. ***P<0.001, Student’st-test. (f,g) Liver tissues were photographed, fixed and stained with haematoxylin and eosin (H&E) (f). Black arrows indicate the liver metastatic lesions; the number of metastatic lesions in each specimen was counted (g). Results are presented as mean±s.d. (n=5). ***P<0.001, Student’st-test. Scale bar, 100 μm. Figure 2: Loss of AF6 promotes tumour proliferation and metastasis. ( a ) Phase-contrast images of Bxpc-3 cells stably expressing control (CT) or either of two AF6 shRNAs and grown as 2D, 3D or 3D invasion cultures (Day 10). Black arrows indicate invasive structures. Scale bar, 100 μm. ( b ) AF6 protein levels in Bxpc-3 cells harbouring control or either of two AF6 shRNAs. ( c ) The sizes of spheroids in a were measured. Data represent the mean±s.d. ( n =30) from three separate experiments. *** P <0.001, Student’s t -test. ( d , e ) Four-week-old nude mice were orthotopically transplanted with Bxpc-3 control (CT) or Bxpc-3 shAF6 cells (shAF6-1 and shAF6-2) (1 × 10 6 cells per animal, n =7); tumours were harvested, photographed ( d ) and weighed at autopsy (Day 60). Results are presented as mean±s.d. ( n =5) of calculated tumour weight ( e ). Scale bar, 1 cm. *** P <0.001, Student’s t -test. ( f , g ) Liver tissues were photographed, fixed and stained with haematoxylin and eosin (H&E) ( f ). Black arrows indicate the liver metastatic lesions; the number of metastatic lesions in each specimen was counted ( g ). Results are presented as mean±s.d. ( n =5). *** P <0.001, Student’s t -test. Scale bar, 100 μm. Full size image Next, we investigated the effects of AF6 on PC proliferation and metastasis in vivo using orthotopic xenograft transplantation of PC cell lines producing either of two AF6 short-hairpin RNAs (shRNAs). We found that at Day 60 post injection, the mean tumour weight was doubled in Bxpc-3 shAF6-implanted animals compared with that in the Bxpc-3-implanted animals. Interestingly, Bxpc-3 shAF6-implanted animals also exhibited a significantly elevated number of micro-metastases in the liver, though not in the lung or spleen ( Fig. 2d–g and Supplementary Fig. 4a ). Conversely, animals implanted with Capan-1 cells harbouring an AF6 forced-expression construct exhibited significant decrease in tumour weight and liver (but not lung or spleen) metastases, compared with those in animals implanted with control cells ( Supplementary Fig. 4b–f ). Thus, these data clearly demonstrated that loss of AF6 expression promotes proliferation and metastasis of PC cells both in vitro and in vivo . AF6 regulates Snail expression To identify possible downstream mediators of AF6’s metastasis suppression effects, we first examined the mRNA levels of the epithelial–mesenchymal transition (EMT) related transcription factors. AF6 downregulation in Bxpc-3 cells was found to cause significant increase in the transcription of Snail and N-cadherin genes, having an opposite effect on that of E-cadherin gene, but scoring almost no effect on those of Slug, Twist , Zeb1 or Zeb2 genes ( Fig. 3a ). Meanwhile, the protein levels of AF6 and Snail were inversely correlated in PC cell lines ( Fig. 3b ). Furthermore, continuously knocking down of AF6 expression in Bxpc-3 or HPAC cells resulted in increased Snail protein levels; conversely, stably overexpressing AF6 in Capan-1 or Capan-2 cells led to marked decrease in the expression level of Snail ( Fig. 3c ). To evaluate whether AF6 regulates Snail transcription, we assayed Snail transcription using a Snail promoter-driven luciferase reporter. We observed that the depletion of AF6 in Bxpc-3 cells resulted in increased reporter expression; in contrast, forced expression of AF6 in Capan-1 or Capan-2 cells led to decreased luciferase production ( Supplementary Fig. 5a ). Taken together, these results suggested that AF6 might negatively regulate the transcription of Snail . 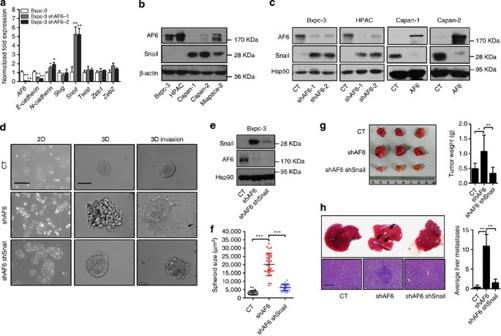Figure 3: Loss of AF6 promotes tumour growth and metastasis via Snail. (a) Real-time PCR analysis of the mRNA expression of the indicated genes in Bxpc-3 or Bxpc-3 shAF6 cells. Data represent the mean±s.d. (n=3) from three separate experiments. *P<0.05, **P<0.01, Student’st-test. (b) Western blot analysis of AF6 and Snail expression in Bxpc-3, HPAC, Capan-1, Capan-2 and Miapaca-2 cells; the protein levels of AF6 and Snail were inversely correlated. (c) Western blot analysis of AF6 and Snail expression in Bxpc-3 and HPAC cells stably transfected with control (CT) or either of twoAF6shRNAs, and in Capan-1 and Capan-2 cells stably transfected with control (CT) or AF6 (AF6)-encoding vectors. (d) Phase-contrast images of Bxpc-3 control (CT), shAF6 and shAF6 shSnail cells grown as 2D, 3D or 3D invasion cultures (Day 10), respectively. Black arrows indicate invasive structures. Scale bars, 100 μm (2D); 50 μm (3D and 3D invasion). (e) Western blot analysis of AF6 and Snail protein levels in cells used ind. (f) The sizes of the spheroids were measured. Data represent the mean±s.d. (n=30) from three independent experiments. ***P<0.001, Student’st-test. (g,h) Four-week-old nude mice were orthotopically transplanted with 1 × 106cells per animal (n=7); tumours were harvested, photographed and weighed at autopsy (Day 60). Results are presented as mean±s.d. (n=7) of calculated tumour weight (g). *P<0.05, **P<0.01, Student’st-test. (h) Liver tissues were photographed, fixed and stained with haematoxylin and eosin (H&E); black arrows indicate the liver metastatic lesions. The number of metastatic lesions in each specimen was counted. Results are presented as mean±s.d. (n=6). **P<0.01, Student’st-test. Scale bar: 100 μm. Figure 3: Loss of AF6 promotes tumour growth and metastasis via Snail. ( a ) Real-time PCR analysis of the mRNA expression of the indicated genes in Bxpc-3 or Bxpc-3 shAF6 cells. Data represent the mean±s.d. ( n =3) from three separate experiments. * P <0.05, ** P <0.01, Student’s t -test. ( b ) Western blot analysis of AF6 and Snail expression in Bxpc-3, HPAC, Capan-1, Capan-2 and Miapaca-2 cells; the protein levels of AF6 and Snail were inversely correlated. ( c ) Western blot analysis of AF6 and Snail expression in Bxpc-3 and HPAC cells stably transfected with control (CT) or either of two AF6 shRNAs, and in Capan-1 and Capan-2 cells stably transfected with control (CT) or AF6 (AF6)-encoding vectors. ( d ) Phase-contrast images of Bxpc-3 control (CT), shAF6 and shAF6 shSnail cells grown as 2D, 3D or 3D invasion cultures (Day 10), respectively. Black arrows indicate invasive structures. Scale bars, 100 μm (2D); 50 μm (3D and 3D invasion). ( e ) Western blot analysis of AF6 and Snail protein levels in cells used in d . ( f ) The sizes of the spheroids were measured. Data represent the mean±s.d. ( n =30) from three independent experiments. *** P <0.001, Student’s t -test. ( g,h ) Four-week-old nude mice were orthotopically transplanted with 1 × 10 6 cells per animal ( n =7); tumours were harvested, photographed and weighed at autopsy (Day 60). Results are presented as mean±s.d. ( n =7) of calculated tumour weight ( g ). * P <0.05, ** P <0.01, Student’s t -test. ( h ) Liver tissues were photographed, fixed and stained with haematoxylin and eosin (H&E); black arrows indicate the liver metastatic lesions. The number of metastatic lesions in each specimen was counted. Results are presented as mean±s.d. ( n =6). ** P <0.01, Student’s t -test. Scale bar: 100 μm. Full size image To investigate whether AF6 modulates tumour progression and metastasis through suppression of Snail expression, we stably knocked down Snail expression in AF6-depleted Bxpc-3 or HPAC cells ( Fig. 3e and Supplementary Fig. 5c ). Indeed, depletion of Snail transcript counteracted the cell morphology changes seen in 2D cell culture, as well as the increased size of spheroid structures and elevated invasive behaviour seen in 3D culturing of cells with AF6 silencing alone ( Fig. 3d,f ; Supplementary Fig. 5b,d and Supplementary Fig. 2a ). Moreover, further depletion of Snail expression in Bxpc-3 shAF6 cells partially restored the expression of E-cadherin ( Supplementary Fig. 2b ). In addition, MTT proliferation and transwell invasion assays confirmed that depletion of Snail reduced cell proliferation and invasion by Bxpc-3 shAF6, HPAC shAF6, Capan-1, Capan-2 and Miapaca-2 cells ( Supplementary Fig. 5e–j ). Furthermore, mice orthotopically implanted with Bxpc-3 shAF6 shSnail cells showed significantly reduced tumour weight and liver metastasis numbers compared with Bxpc-3 shAF6-implanted animals ( Fig. 3g,h ). We also found that mice implanted with Capan-1 shSnail cells showed significant attenuation of tumour weight and of liver (but not lung or spleen) metastases compared with Capan-1 implanted animals ( Supplementary Fig. 4b–f ). Collectively, these data implied that Snail is a key downstream effector of the enhanced in vivo tumour growth and metastasis seen on loss of AF6 expression. Nuclear AF6 is required to repress Snail expression Accumulating evidence suggests that AF6 is a dual-residency protein, and its nuclear localization and transcriptional repressor activity are closely correlated [14] , [24] , [25] , [26] . As shown in Fig. 4a and Supplementary Fig. 6a , immunofluorescence analysis indicated that AF6 was located in both the cell membrane and the nucleus in Bxpc-3 and HPAC cells. All of the immunofluorescence staining was abrogated when AF6 was knocked down, thus excluding the possible cross-reactivity by the anti-AF6 antibodies. Consistently, our subcellular fractionation experiments further indicated that a fraction of AF6 was indeed localized in nuclear ( Fig. 4b and Supplementary Fig. 6b ). We further tested the role of a nuclear localization sequence (NLS) known to promote protein nuclear translocation. We found that expression of NLS–AF6 repressed Snail expression; in contrast, expression of ΔNLS–AF6, a NLS-deleted form of AF6, abolished the repressive effect of AF6 on the expression of Snail ( Fig. 4c,d ). Collectively, these data suggested that the nuclear localization of AF6 is required for its repression of Snail expression. 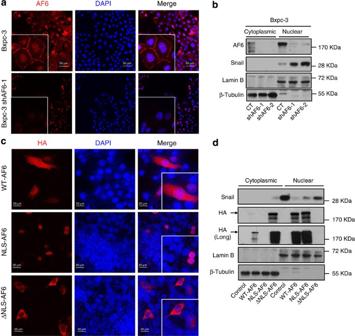Figure 4: Nuclear localized AF6 is required to repressSnailexpression. (a) Wild-type and Bxpc-3 shAF6 cells were immunostained with AF6 (red) or DAPI (blue). Scale bars, 50 μm. (b) Western blot analysis of AF6 and Snail expression in cytoplasmic and nuclear extracts derived from control (CT) and Bxpc-3 shAF6 cells (shAF6-1 and shAF6-2). (c) Capan-1 cells seeded in 35-mm dishes were transiently transfected with 500 ng of HA–WT-AF6 (WT-AF6), HA–NLS–AF6 (NLS–AF6) or HA–ΔNLS–AF6 (ΔNLS–AF6) plasmids; localization of AF6 was detected by immunofluorescence (IF) analysis of HA (red) and DAPI (blue). Scale bars, 20 μm. (d) Western blot analysis of AF6 and Snail expression in cytoplasmic and nuclear extracts derived from Capan-1 cells transiently transfected with control empty vector (Control), HA–WT-AF6 (WT-AF6), HA–NLS–AF6 (NLS–AF6) or HA–ΔNLS–AF6 (ΔNLS–AF6) plasmids, blank arrows indicate AF6; long, long exposure. Figure 4: Nuclear localized AF6 is required to repress Snail expression. ( a ) Wild-type and Bxpc-3 shAF6 cells were immunostained with AF6 (red) or DAPI (blue). Scale bars, 50 μm. ( b ) Western blot analysis of AF6 and Snail expression in cytoplasmic and nuclear extracts derived from control (CT) and Bxpc-3 shAF6 cells (shAF6-1 and shAF6-2). ( c ) Capan-1 cells seeded in 35-mm dishes were transiently transfected with 500 ng of HA–WT-AF6 (WT-AF6), HA–NLS–AF6 (NLS–AF6) or HA–ΔNLS–AF6 (ΔNLS–AF6) plasmids; localization of AF6 was detected by immunofluorescence (IF) analysis of HA (red) and DAPI (blue). Scale bars, 20 μm. ( d ) Western blot analysis of AF6 and Snail expression in cytoplasmic and nuclear extracts derived from Capan-1 cells transiently transfected with control empty vector (Control), HA–WT-AF6 (WT-AF6), HA–NLS–AF6 (NLS–AF6) or HA–ΔNLS–AF6 (ΔNLS–AF6) plasmids, blank arrows indicate AF6; long, long exposure. Full size image Loss of AF6 induces Snail expression via Dvl2 Prior work suggested that reduced AF6 expression led to activation of Erk1/2 and Src, as well as enhanced migratory and proliferative phenotype of breast cancer cells [13] . To identify possible downstream mediators of AF6’s repressive effect on Snail expression, we first determined whether loss of AF6 induced Snail expression through activation of Erk1/2 and Src in PC cells. Notably, depletion of AF6 in Bxpc-3 or HPAC cells did not lead to activation of Erk1/2 or Src ( Supplementary Fig. 7a ), suggesting the existence of alternative mechanisms in regulating Snail gene expression by AF6. A previous report demonstrated that Canoe/AF6 interacts with Dvl, which is essential for the cross-communication of the Ras-MAPK, Notch and wnt signalling pathways in Drosophila [27] . Dvl2, an isoform of Dvl, also has been reported to contribute to PC malignancy through stabilization of β-catenin [28] . We speculated that Dvl2 might mediate the induction of Snail expression on loss of AF6 in PC cells. To test this hypothesis, we first assessed the interaction between AF6 and Dvl2 in PC cells. Indeed, endogenous AF6 formed complex with Dvl2 in both Bxpc-3 and HPAC cells ( Fig. 5a ). In addition, AF6 also interacts with all three Dvl isoforms of the human Dvl family ( Supplementary Fig. 7b ). As shown in Fig. 5b,c , overexpression of Dvl2 in 293T cells increased transcription of Snail gene, and the static level of Snail protein as well. Luciferase-based reporter assay further indicated that overexpression of AF6 inhibited Snail transcription, through antagonizing Dvl2-induced Snail promoter transactivation ( Fig. 5d ). Moreover, continuously knocking down of Dvl2 in Capan-1, Capan-2, Miapaca-2, Bxpc-3 shAF6 and HPAC shAF6 cells demonstrated that decrease in Dvl2 expression was associated with reductions in the static levels of Snail protein, cell proliferation and cell invasion ( Fig. 5e–g and Supplementary Fig. 7c–e ), reminiscent of the effect of Snail deficiency ( Supplementary Fig. 5e–j ). In addition, we demonstrated that depletion of AF6 expression in Bxpc-3 or HPAC cells did not change β-catenin protein levels ( Supplementary Fig. 7a ), thus excluding the possibility that Dvl2 regulates Snail expression through the canonical Wnt-β-catenin pathway. Altogether, these results indicated that loss of AF6 induces Snail expression through Dvl2. 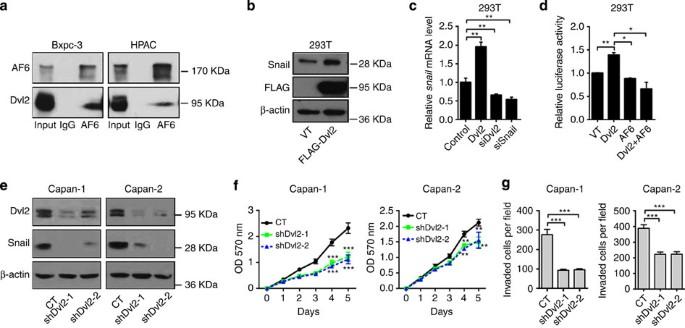Figure 5: Loss of AF6 induces Snail expression via Dvl2. (a) Endogenous AF6 bound to endogenous Dvl2 in Bxpc-3 and HPAC cells. Cell lysates from confluent monolayers of Bxpc-3 or HPAC cells were immunoprecipitated using anti-AF6 and immunoblotted as indicated. (b) Dvl2 induces Snail protein expression. 293T cells transiently transfected with control empty (VT) or FLAG–Dvl2 vectors were analysed by Western blot. (c) Real-time PCR analysis of expression ofSnailin 293T cells transiently transfected with control empty vector (Control); with FLAG–Dvl2 plasmids; withDvl2siRNAs; or withSnailsiRNAs. Data represent the mean±s.d. (n=3) from three separate experiments. **P<0.01, Student’st-test. (d) 293T cells were transfected with empty vector (VT); FLAG–Dvl2 plasmids; HA–AF6 plasmids; or constructs encoding both Dvl2 and AF6. At 48 h post transfection, cells were assayed forSnailpromoter-driven luciferase activity. Results are presented as mean±s.d. (n=3) from three independent experiments. *P<0.05, **P<0.01, Student’st-test. (e) Dvl2 and Snail protein level in Capan-1 or Capan-2 cells stably expressing control shRNA (CT) or twoDvl2shRNAs. (f) MTT proliferation assay in control orDvl2shRNA-expressing Capan-1 or Capan-2 cells. Data represent the mean±s.d. (n=3) from three independent experiments. **P<0.01, ***P<0.001, Student’st-test. (g) Transwell invasion assay for control orDvl2shRNA-expressing Capan-1 or Capan-2 cells. Data represent the mean±s.d. (n=3) from three independent experiments. ***P<0.001, Student’st-test. Figure 5: Loss of AF6 induces Snail expression via Dvl2. ( a ) Endogenous AF6 bound to endogenous Dvl2 in Bxpc-3 and HPAC cells. Cell lysates from confluent monolayers of Bxpc-3 or HPAC cells were immunoprecipitated using anti-AF6 and immunoblotted as indicated. ( b ) Dvl2 induces Snail protein expression. 293T cells transiently transfected with control empty (VT) or FLAG–Dvl2 vectors were analysed by Western blot. ( c ) Real-time PCR analysis of expression of Snail in 293T cells transiently transfected with control empty vector (Control); with FLAG–Dvl2 plasmids; with Dvl2 siRNAs; or with Snail siRNAs. Data represent the mean±s.d. ( n =3) from three separate experiments. ** P <0.01, Student’s t -test. ( d ) 293T cells were transfected with empty vector (VT); FLAG–Dvl2 plasmids; HA–AF6 plasmids; or constructs encoding both Dvl2 and AF6. At 48 h post transfection, cells were assayed for Snail promoter-driven luciferase activity. Results are presented as mean±s.d. ( n =3) from three independent experiments. * P <0.05, ** P <0.01, Student’s t -test. ( e ) Dvl2 and Snail protein level in Capan-1 or Capan-2 cells stably expressing control shRNA (CT) or two Dvl2 shRNAs. ( f ) MTT proliferation assay in control or Dvl2 shRNA-expressing Capan-1 or Capan-2 cells. Data represent the mean±s.d. ( n =3) from three independent experiments. ** P <0.01, *** P <0.001, Student’s t -test. ( g ) Transwell invasion assay for control or Dvl2 shRNA-expressing Capan-1 or Capan-2 cells. Data represent the mean±s.d. ( n =3) from three independent experiments. *** P <0.001, Student’s t -test. Full size image FOXE1 trans -activates Snail expression Though AF6 or Dvl2 regulates Snail expression at the transcriptional level, neither AF6 nor Dvl2 is a transcription factor. We therefore speculated that a transcription factor might be involved, potentially through direct interaction with both AF6 and Dvl2. An haemagglutanin (HA)-tag affinity procedure was used to purify an AF6-containing complex from 293T cells, followed by mass spectrometric analysis. Peptide sequences for FOXE1, a member of mammalian forkhead box (FOX) family of transcription factors [29] , were recovered, suggesting that FOXE1 is present in the AF6-containing complex ( Supplementary Fig. 8a ). Co-immunoprecipitation (co-IP) experiment further indicated that endogenous AF6 did form a complex with FOXE1 in Bxpc-3 cells ( Fig. 6a ). Furthermore, we found that forced expression of FOXE1 in 293T cells induced Snail protein production ( Fig. 6b ). In silico analysis of the Snail promoter (the 1,500 bp upstream of the Snail +1 transcription start site) revealed the presence of three putative FOXE1 consensus binding sites [30] (AAACA, located at −1405 to −1401, −1319 to −1315, and −623 to −619) ( Supplementary Fig. 8b ). Chromatin IP (ChIP) assay revealed that FOXE1 directly bound to the start site-distal binding site of the Snail promoter ( Supplementary Fig. 8c ). The luciferase reporter assay also showed that FOXE1 trans -activates Snail promoter activity; mutation (from AAACA to TCTT) in the start site-distal FOXE1-binding site significantly decreased FOXE1-induced activity ( Supplementary Fig. 8d ). These results indicated that FOXE1 is a direct transcriptional regulator of Snail . 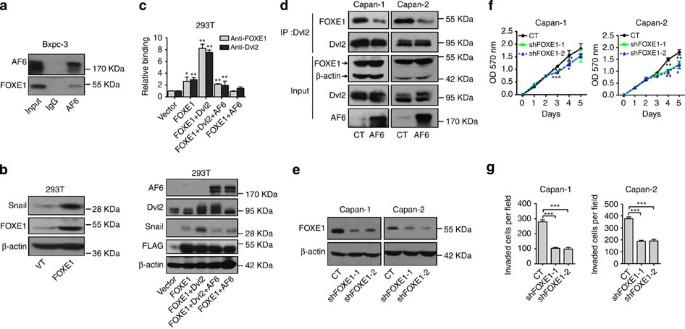Figure 6: AF6 antagonizes Dvl2- and FOXE1-mediatedSnailtransactivation. (a) Endogenous AF6 bound to endogenous FOXE1 in Bxpc-3 cells. Cell lysates from confluent monolayers of Bxpc-3 cells were immunoprecipitated using anti-AF6 and immunoblotted as indicated. (b) Western blot analysis of Snail protein expression from 293T cells transfected with an empty vector (VT) or with a construct encoding FOXE1. (c) 293T cells were transfected with the indicated plasmids, and cultures were analysed for FOXE1 or Dvl2 binding to theSnailpromoter (upper) or for Snail protein expression (lower). Data represent the mean±s.d. (n=3) from three independent experiments. *P<0.05, **P<0.01, Student’st-test. (d) AF6 attenuates the interaction between FOXE1 and Dvl2. Capan-1 or Capan-2 cells were stably transfected with a control empty vector (CT) or an AF6-encoding plasmid (AF6); cell lysates were subjected to IP and western blot analyses. (e) FOXE1 protein level in Capan-1 or Capan-2 cells stably expressing control shRNA (CT) or twoFOXE1shRNAs. (f) MTT proliferation assay in Capan-1 or Capan-2 cells expressing control orFOXE1shRNAs. Data represent the mean±s.d. (n=3) from three independent experiments. *P<0.05, **P<0.01, ***P<0.001, Student’st-test. (g) Transwell invasion assay for control orFOXE1shRNA-expressing Capan-1 or Capan-2 cells. Data represent the mean±s.d. (n=3) from three independent experiments. ***P<0.001, Student’st-test. Figure 6: AF6 antagonizes Dvl2- and FOXE1-mediated Snail transactivation. ( a ) Endogenous AF6 bound to endogenous FOXE1 in Bxpc-3 cells. Cell lysates from confluent monolayers of Bxpc-3 cells were immunoprecipitated using anti-AF6 and immunoblotted as indicated. ( b ) Western blot analysis of Snail protein expression from 293T cells transfected with an empty vector (VT) or with a construct encoding FOXE1. ( c ) 293T cells were transfected with the indicated plasmids, and cultures were analysed for FOXE1 or Dvl2 binding to the Snail promoter (upper) or for Snail protein expression (lower). Data represent the mean±s.d. ( n =3) from three independent experiments. * P <0.05, ** P <0.01, Student’s t -test. ( d ) AF6 attenuates the interaction between FOXE1 and Dvl2. Capan-1 or Capan-2 cells were stably transfected with a control empty vector (CT) or an AF6-encoding plasmid (AF6); cell lysates were subjected to IP and western blot analyses. ( e ) FOXE1 protein level in Capan-1 or Capan-2 cells stably expressing control shRNA (CT) or two FOXE1 shRNAs. ( f ) MTT proliferation assay in Capan-1 or Capan-2 cells expressing control or FOXE1 shRNAs. Data represent the mean±s.d. ( n =3) from three independent experiments. * P <0.05, ** P <0.01, *** P <0.001, Student’s t -test. ( g ) Transwell invasion assay for control or FOXE1 shRNA-expressing Capan-1 or Capan-2 cells. Data represent the mean±s.d. ( n =3) from three independent experiments. *** P <0.001, Student’s t -test. Full size image AF6 inhibits Dvl2/FOXE1 complex-mediated Snail transcription As AF6 interacts both with Dvl2 and FOXE1, it is intriguing to ask whether Dvl2 and FOXE1 interact with each other. Indeed, Dvl2 interacted with both AF6 and FOXE1 in 293T cells as assessed by co-IP assay ( Supplementary Fig. 9a ). It is remains to be seen whether AF6 and Dvl2 might exert opposite effect on Snail gene expression through direct competing with each other in the interaction with FOXE1. To test this possibility, ChIP analyses were carried out. On AF6 depletion, more FOXE1 or Dvl2 was recruited to the Snail promoter, compared with that in control cells ( Supplementary Fig. 9b ). Furthermore, forced expression of Dvl2 in FOXE1 -overexpressing 293T cells resulted in increased FOXE1 and Dvl2 recruitment to the Snail promoter, along with marked increase in static level of Snail protein. Interestingly, such effect could be reversed by AF6 overexpression ( Fig. 6c ). In addition, we found that overexpression of AF6 or knockdown of FOXE1 or Dvl2 alone resulted in decreased recruitment of FOXE1 and Dvl2 to the Snail promoter ( Supplementary Fig. 9c ). Furthermore, MTT proliferation and transwell invasion assays revealed that knockdown of FOXE1 attenuated the proliferative and invasive activities in a manner similar to that seen on knockdown of Dvl2 ( Fig. 6e–g and Supplementary Fig. 10a–c ). Taken together, these results demonstrated that the increased cell proliferation and invasion phenotype seen on depletion of AF6 is mediated primarily through Dvl2-regulated recruitment of FOXE1 to increase Snail transcription. Negative correlation of AF6 and Snail in clinical samples To determine the relevance of our experimental findings to the pathogenesis of human PC, we first examined the expression pattern of Snail, Dvl2, FOXE1 and AF6 in 31 human PDAC samples. Notably, IHC analyses revealed that Snail expression is negatively correlated with AF6 expression and positively correlated with Dvl2 and FOXE1 expression in human PC ( Supplementary Fig. 11 and Supplementary Table 1 ). We further investigated the correlation of AF6 and Snail expression with clinical features of pancreatic tumours. Kaplan–Meier analysis of specimens from 83 human PDAC patients showed that patients harbouring tumours with high AF6 protein levels ( n =30; median survival time=23.5 months) had longer overall survival times than patients harbouring tumours with low AF6 protein levels ( n =53; median survival time=10 months; P <0.05) ( Fig. 7a ). Consistent with this result, patients harbouring tumours with low Snail protein levels ( n =27; median survival time=31 months) had longer overall survival times than those harbouring tumours with high Snail protein levels ( n =56; median survival time=10 months; P <0.01) ( Fig. 7b ). In addition, correlation analyses revealed that in 158 human PC samples, 109 (69.0%) samples exhibited low AF6 expression levels; of these, 63 (57.8%) samples displayed elevated Snail expression ( Supplementary Fig. 12a ). Furthermore, in silico pairwise correlation analyses of the mRNA expression levels of AF6 and Snail in three independent data sets obtained from Oncomine confirmed an inverse correlation in human PC, as well as in normal pancreas or PanINs ( Supplementary Fig. 12b ). Moreover, the decreased level of AF6 or increased level of Snail transcript was associated with larger tumour size and higher tumour grade level in patients ( Supplementary Table 2 ). These clinical findings indicated that low expression level of AF6 may be related to high Snail expression level and malignant progression of PC. 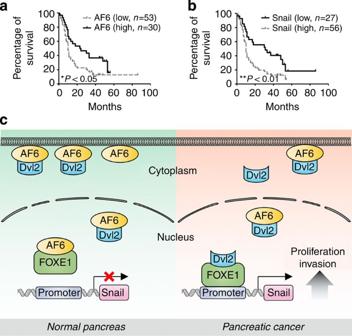Figure 7: The levels of AF6 and Snail expression in pancreatic cancer have prognostic implications. (a) Kaplan–Meier curves for overall survival in 83 human pancreatic cancer patients classified by relative (high or low) immune signal for AF6 and Snail protein levels. The log-rank (Mantel-Cox) testPvalue reflects the significance of the correlation between AF6 positivity or Snail negativity and longer survival outcomes. *P<0.05, **P<0.01, log-rank test. (b) Model of the role of AF6 in normal pancreas and in pancreatic cancer. Figure 7: The levels of AF6 and Snail expression in pancreatic cancer have prognostic implications. ( a ) Kaplan–Meier curves for overall survival in 83 human pancreatic cancer patients classified by relative (high or low) immune signal for AF6 and Snail protein levels. The log-rank (Mantel-Cox) test P value reflects the significance of the correlation between AF6 positivity or Snail negativity and longer survival outcomes. * P <0.05, ** P <0.01, log-rank test. ( b ) Model of the role of AF6 in normal pancreas and in pancreatic cancer. Full size image Thus, our studies demonstrated that AF6 can inhibit proliferation and metastasis of PC cells, with its acting through the Dvl2–FOXE1–Snail axis. A proposed model is summarized schematically in Fig. 7c . In normal pancreas, AF6 is abundantly expressed and located both in the cell membrane and nucleus; Dvl2 is kept at low expression levels; and AF6 represses Snail transcription by antagonizing the interaction between FOXE1 and Dvl2. In PC cells, AF6 is expressed at low levels; conversely, Dvl2 is upregulated. Dvl2 then is available to bind and enhance FOXE1-induced trans -activation of Snail , which further promotes proliferation and metastasis of PC cells. As reported here, the cell polarity protein AF6 is expressed at low levels in the majority of human pancreatic adenocarcinomas and PC precursor lesions. Loss of AF6 in PC cells promotes cellular proliferation, tumour growth and metastasis, as measured both by in vitro and in vivo assays. Moreover, depletion of AF6 induces transcription of Snail in cell lines and in primary PCs, and knockdown of Snail largely prevents the tumour growth and metastasis associated with loss of AF6. We additionally demonstrated that the effect of AF6 depletion on Snail expression is mediated by protein–protein interactions between AF6 and Dvl2, which in turn affect FOXE1 binding and transcription at the Snail promoter. Furthermore, we showed that Snail protein levels negatively correlate with the protein levels of AF6 and positively correlate with the protein levels of Dvl2 and FOXE1 in clinical PC samples, and that the patients with higher AF6 or lower Snail protein levels exhibit longer overall survival times. In summary, our studies suggest that AF6 is a potential inhibitor of the metastasis of PC cells, a regulatory effect that is mediated through the Dvl2–FOXE1–Snail axis. Our study provides new insights into how cell polarity protein AF6 serves as an important negative regulator by suppressing expression of the EMT inducer Snail in PC. The EMT is an essential process governing morphogenesis in multicellular organisms and its activation can lead to metastasis of primary tumours during the progression of carcinoma [31] . One of the earliest steps in EMT is the loss of cell–cell adhesion and disruption of apical-basal cell polarity, as well as increased motility of cells. In migrating cells, polarity proteins are important regulators of front-back polarity; many cell polarity proteins (including Scribble, Par3 and Par6) are localized to the leading edge of migrating cells and play important roles during directional migration [32] . Migration of cells is associated with changes in cell architecture, suggesting that cell polarity proteins play important roles during this process. Recently, the polarity protein Par6 has been shown to play a critical role during TGFβ-induced EMT [33] , [34] . In addition, loss of Hugl-1 also is associated with EMT in melanoma cells; restoration of expression Hugl-1 restores epithelial cell polarity while also inhibiting cell migration [35] . These studies suggest that cell polarity has a close relationship with the EMT process during the progression of cancer. EMT inducers, such as Snail, Twist, Slug and Zeb1/2, previously have been shown to drive a transcriptional programme that transforms epithelial cells to potentially aggressive cancer cells. Snail is a conserved transcription factor that has been shown to play an important role in embryonic development and tumour progression [36] . Extensive analysis of such EMT inducers has clearly demonstrated a role in the direct regulation of cell polarity genes at the transcription level, contributing to the progression of cancer [37] . However, little information exists regarding the feedback regulation of these EMT inducers by cell polarity signalling. Interestingly, the present work showed that the cell polarity protein AF6 can directly repress Snail transcription in pancreatic cells. Our observations suggest how aberrant polarity signalling can promote the process of tumorigenicity by direct regulation of EMT inducers in cancer cells. The roles of cell polarity proteins appear to be much more complex than scaffolding functions at the defined sites, instead involving intracellular signalling and gene expression. It will be interesting to elucidate the multiple functions and the dynamic aspects of cell polarity proteins in the nucleus. Intriguingly, we found that AF6 represses Snail expression depending on AF6’s nuclear localization in PC cells. A similar phenomenon of AF6 nuclear localization also was observed when cells were exposed to growth factor signalling, and nuclear localization of AF6 may facilitate the induction of a transcriptional programme [14] , [24] , [25] , [26] . However, there exists little evidence to show that AF6 can play a role as a transcriptional co-factor. Surprisingly, we found that AF6 directly interacts with transcription factor FOXE1 and functions as a transcriptional co-factor to repress Snail transcription. These findings may provide a potential new approach for investigating the role of cell polarity proteins implicated in gene expression and regulation in the nucleus. A larger question that still needs to be explored is that how AF6 is lost during the development of PC. To investigate whether downregulation of AF6 resulted from promoter hypermethylation or post-translational proteasomal degradation, we performed the following two studies. (1) In one study, we treated Capan-1 and Capan-2 (PC cell lines that harbour relatively low endogenous level of AF6 expression) with different concentrations of 5-Aza-dcr, a DNA methyltransferase inhibitor, and examined effects on the mRNA expression level of AF6. (2) In a second study, we treated Capan-1 and Capan-2 cell lines with MG132, a proteasome inhibitor, examined effects on the protein expression level of AF6. We found that neither treatment resulted in the induction of AF6 expression ( Supplementary Fig. 13a,b , respectively). Together, these results suggested that downregulation of AF6 in PC was not due to promoter hypermethylation or post-translational proteasomal degradation, implying that other underlying mechanisms are involved in this process. We propose to make this topic the subject of future work in our laboratory. Our observations also demonstrate a novel perspective on the role played by the AF6–Dvl2–FOXE1 axis in regulating the transcription of Snail . Surprisingly, we found that the induction of Snail expression by decreasing AF6 expression was mediated primarily via Dvl2. Emerging work suggests that Dvl2 plays an important role in the nuclear regulation of gene expression [38] , [39] , [40] . Further analysis identified FOXE1, a transcription factor, as a binding partner of AF6. The FOXE1 gene has been shown to be aberrantly methylated in PC [41] , [42] . However, the function of FOXE1 during PC tumorigenesis has yet to be investigated. Interestingly, we found that Dvl2 could interact with FOXE1 to increase the trans -activation of Snail by a mechanism independent of the canonical Wnt-β-catenin signalling pathway; this increase in Snail transcription was impaired in the presence of AF6, presumably via inhibition of the binding between FOXE1 and Dvl2. These results reveal the existence of a novel regulatory complex (containing AF6, Dvl2 and FOXE1) that mediates Snail transcriptional regulation in PC cells, shedding new light on cross-talk among cell polarity proteins, Dvl proteins and FOX family proteins. These results also suggest a potential new research target (the regulation of FOX proteins by Dvl proteins) that could have broad implications in development and cancer progression. In conclusion, our analyses have demonstrated that AF6, as a negative regulator of Snail , serves as a potential suppressor in the progression and metastasis of PC. Notably, our data may provide a potential new direction to investigate the role of cell polarity proteins implicated in gene expression and regulation during tumorigenesis. Indeed, these findings will surely improve our understanding of the diverse functions and mechanisms of action of cell polarity proteins, and also define AF6 as a potential target for early detection or therapeutic intervention in PC progression. Tumour samples This study was approved by the Institutional Review Board of the Institute for Nutritional Sciences, Chinese Academy of Sciences. Three validated cohorts of patients with informed written consent were used in the study. The first cohort consisted of 40 PC patients, from whom tumour specimens were obtained at the time of surgical resection from Changhai Hospital (The Second Military Medical University, China). These specimens were used for real-time PCR analysis. Differentiation status of members of this cohort are listed in Supplementary Table 3 . The second cohort consisted of 31 patients from whom specimens were obtained as tissue microarray (TMA) chips from the Biobank Center of National Engineering Center for Biochip at Shanghai (also known as Shanghai Outdo Biotech Company, Ltd). The TMA specimens were used for IHC analysis. The third cohort used for correlation analysis consisted of 158 cases, from whom specimens also were obtained as TMA chips from the Biobank Center of National Engineering Center for Biochip. The TMA specimens were used for IHC analysis. About 90 cases used for IHC score analysis and 83 cases used for Kaplan–Meier survival analysis were included in this cohort. TMA construction Pancreatic TMAs were constructed using tissue cores from formalin-fixed, paraffin-embedded specimens as described previously [43] . Briefly, representative tumour areas and corresponding non-tumour pancreatic specimens were selected by pathologists from each tissue block, and then a single core with a diameter of 1.5 mm was taken from each case. Microarray blocks were constructed by using an automated tissue arrayer (Beecher Instruments, Sun Prarie, WI). Five-micron sections were cut from the array blocks, then sections were stained with haematoxylin and eosin to verify the presence of tumour cells. In all cases, tissue cores obtained from normal adjacent pancreas served as internal controls. Cell culture and transfection Bxpc-3, Aspc-1, CFPAC-1, Capan-1, Capan-2, SW1990, Miapaca-2, PANC-1, 293T and HPAC cells were obtained from the American Type Culture Collection (Manassas, VA) and grown in DMEM medium (Life Technologies) supplemented with 10% foetal bovine serum (Hyclone) and 1% penicillin/streptomycin (Life Technologies). MCF-10A cells, also obtained from ATCC, were grown in DMEM/F12 medium (Life Technologies) supplemented with 5% horse serum (Life Technologies), 20 ng ml −1 epidermal growth factor (R&D), 10 μg ml −1 insulin (Sigma), 0.5 μg ml −1 hydrocortisone (Sigma), 100 ng ml −1 cholera toxin (Sigma) and 1% penicillin/streptomycin. HPDE cells (provided by Dr Ming-Sound Tsao, the Ontario Cancer Institute, Toronto, ON, Canada) were grown in a keratinocyte serum-free medium supplemented with 5 ng ml −1 epidermal growth factor and 50 μg ml −1 bovine pituitary extract (Life Technologies). For all cultures, cells were incubated at 37 °C in a humidified atmosphere with 5% CO 2 . Transfection of the plasmids and siRNAs into the cells was conducted using Lipofectamine 2,000 reagent (Life Technologies) according to the manufacturer’s protocol. Antibodies and reagents Antibodies and reagents were obtained as follows: anti-AF6 antibody (western blot (WB), 1:1,000; IP, 1:400) from BD Transduction Laboratories or Abcam Company; anti-FOXE1 (WB, 1:2,000; IP, 1:800) antibody from Abcam Company; anti-Hsp90 (WB, 1:1,000), anti-Snail (WB, 1:1,000), anti-Dvl2 (WB, 1:1,000; IP, 1:400) and anti-HA (WB, 1:2,000; IP, 1:400) antibodies and horseradish peroxidase-conjugated secondary antibodies from Cell Signaling Technology (WB, 1:1,000); anti-GAPDH (WB, 1:1,000) and anti-β-actin (WB, 1:1,000) antibodies from Abmart Company; anti-myc (WB, 1:1,000; IP, 1:400) and all siRNAs from Santa Cruz Biotechnology, Inc.; anti-FLAG (WB, 1:1,000; IP, 1:400) antibody from Sigma-Aldrich; collagen-I and Matrigel from BD Pharmingen. Immunohistochemistry was performed using primary antibodies against AF6 (1:250, Sigma), Dvl2 (1:250, Millipore), Snail (1:250, Thermo Scientific), and FOXE1 (1:400). Plasmids l-afadin- and s-afadin-encoding plasmids were kindly provided by Dr M. Meyer zu Brickwedde (the University of Muenster, Germany); HA–AF6- and Myc–AF6-encoding gene sequences were synthesized and cloned into the pEF-BOS vector [44] ; plasmids encoding FLAG–Dvl1 and FLAG–Dvl3 were generously provided by Dr Lin Li (SIBCB, China); a plasmid encoding FLAG–Dvl2 was kindly provided by Dr Yue-Zhen Deng (INS, China). The complementary DNA open reading frame encoding human FOXE1 was obtained from a FLAG–FOXE1-encoding vector (Origene) and cloned into pCMV-C-HA (Beyotime) using EcoRI–XbaI restriction sites. The wild-type and mutant Snail promoters (−1,500 to +1) were synthesized and cloned into the pGL 3.0 basic vector (Promega) using KpnI–XhoI restriction sites. The ΔNLS–AF6 plasmid was generated by deletion of the codons encoding the NLS (amino acids ERKRRE) from AF6 (as derived from the HA–AF6 plasmid); the NLS–AF6 plasmid was generated through insertion of three copies of the NLS-encoding sequence (derived from pHcRed1-Nuc vector; Clontech Laboratories, Inc.) at the downstream end of the AF6 open reading frame (as derived from the HA–AF6 plasmid). Plasmid constructions and PCR were performed using standard molecular biology techniques. RNAi sequences were designed using the shRNA library of the RNAi Codex (codex.cshl.edu). The AF6 short-hairpin RNAi, which consists of a 116-base oligonucleotide with flanking sites, was synthesized and cloned into the pMSCV PIG (Puro IRES GFP) retroviral expression vector (Addgene) using flanking XhoI and EcoRI restriction sites (underlined below). The sense sequences were as follows: shAF6-1 : 3′-CTCGAGAAGGTATATTGCTGTTGACAGTGAGCGCGGTGGAACATTGAGAATTTATTAGTGAAGCCACAGATGTAATAAATTCTCAATGTTCCACCTTGCCTACTGCCTCGGAATTC-5′; shAF6-2 : 3′-CTCGAGAAGGTATATTGCTGTTGACAGTGAGCGAGGCGTCCCATGTATTTAAGTTTAGTGAAGCCACAGATGTAAACTTAAATACATGGGACGCCCTGCCTACTGCCTCGGAATTC-5′. pGIPZ Snail lentiviral short-hairpin RNA vectors were purchased from Thermo Scientific. The Dvl2 and FOXE1 short-hairpin RNAi were synthesized and cloned into the lentiviral GV248 vector (Genechem, China). The targeted sequences were as follows: sh Dvl2-1 : 3′-TGTAGCTGCCTTTGTTACTCTATTTATTT-5′; shDvl2-2: 3′-GGACCGCATGTGGCTCAAGATCACCATCC-5′; sh FOXE1-1 : 3′-CCTTTAACTGCGTTACTACAA-5′; sh FOXE1-2 : 3′-CATCTACAAGTTCATCACCGA-5′ Lentiviral virus preparation, infection and selection were performed according to the vector’s technical manual. Stable cell-line construction Retrovirus was produced by transiently transfecting the 293-GPG packaging cells seeded in 10 cm dishes with 12 μg of pMSCV PIG AF6 shRNA vector; 2 days after transfection viral supernatant was collected, filtered and added to the Bxpc-3 or HPAC cells. After 2 days, cells were selected with 2 μg ml −1 puromycin for 2 weeks. Stable AF6-overexpressing Capan-1 and Capan-2 cell lines were generated using lentiviral vector pRRL-AF6FL; this vector, which encodes full-length AF6, was generously provided by Dr M Lopez (University of the Mediterranee, Marseille, France). Lentivirus production and cell-line constructions were performed as described previously [45] ; in brief, the virus particles were produced by transient transfection into 293T cells seeded in 6-cm dishes with 2.7 μg of the packaging construct, 0.9 μg of the construct that express the vesicular stomatitis virus glycoprotein and 2.7 μg of the pRRL-AF6FL vector, and the media from the transfected cells was collected as the cells were re-fed each day for 3–4 days. The virus-containing media was pooled, filtered and used to generate AF6-overexpressing stable cell lines. 3D cell culture and invasion assay For 3D cell culture, 4,000 cells were seeded onto 8-well chamber slides coated with 70 μl per well of Matrigel and fresh media containing matrigel was added every 3 days. For the 3D invasion assay, cells were seeded at 4,000 cells per well in 8-well chamber slides (Thermo Scientific) coated with 70 μl per well of Matrigel-collagen matrix (1.0 ml Matrigel, 1.0 ml Collagen-I, 125 μl 10 × phosphate-buffered saline (PBS), 125 μl NaOH, 25 μl of 0.1 mol l −1 HCl). Phase images were captured on an IX51 Microscope (Olympus). The cell size measurement was calculated by ImageJ. Nuclear and cytoplasmic protein extraction Nuclear and cytoplasmic proteins were extracted using NE-PER Nuclear and Cytoplasmic Extraction Reagents (Thermo Scientific) according to the manufacturer’s protocol. Briefly, cells were harvested by adding typsin-EDTA, washed with ice-cold PBS and then lysed in ice-cold CER I for 15 min, followed by addition of ice-cold CER II and incubation on ice for 1 min. Cells then were centrifuged at 16,000 g for 5 min and the supernatant containing the cytoplasmic proteins was removed and stored for use. The insoluble pellet was re-suspended in ice-cold NER and incubated on ice for 40 min. The resulting suspensions were centrifuged at 16,000 g for 10 min, and the resulting supernatant (containing the nuclear proteins) was recovered and stored at −20 °C pending analysis. WB and IP For WB, cells were collected and lysed in RIPA buffer (Cell Signaling), then centrifuged at 12,000 g for 10 min at 4 °C. The supernatant was recovered and protein concentration was assessed using the Bio-Rad protein assay kit (Bio-Rad, Hercules, CA) according to the manufacturer’s protocol. Identical amounts of protein were subjected to SDS–PAGE electrophoresis and transferred to pre-activated polyvinylidene fluoride membranes (Millipore). The blotted membranes were blocked with 5% fat-free milk for 1 h at room temperature and incubated overnight with primary antibodies at 4 °C, then with secondary antibodies for 1.5 h at room temperature. Finally, the bands were visualized using the ECL chemiluminescence kit (Pierce). For IP, Bxpc-3 and HPAC cells or 293T cells transfected with indicated plasmids were washed with ice-cold PBS, pelleted and lysed in IP lysis buffer (Pierce) for 10 min at 4 °C, and centrifuged at 12,000 g for 10 min at 4 °C. The supernatant was recovered and incubated overnight at 4 °C with the corresponding primary antibody. Protein G Sepharose beads (Amersham/GE) were added and further incubated for 4 h at 4 °C; the beads then were washed three times with Tris-buffered saline and boiled for 5 min in 100 μl of 2 × SDS loading buffer. Representative original images of immunoblotting results for Figs 1 , 2 , 3 , 4 , 5 , 6 are shown in Supplementary Fig. 14 . RNA extraction and real-time PCR Total RNA was extracted using TRIzol reagent (Invitrogen). RNA was reverse transcribed with PrimerScript RT–PCR Kit (Takara) to generate complementary DNA for real-time PCR using SYBR Premix Ex Taq (Takara) in an CFX96 Real-Time PCR Detection System (Bio-Rad). Primers used for real-time PCR are shown in Supplementary Table 4 . Oncomine data analyses Oncomine data analyses were performed as previously described [46] . Briefly, we searched for MLLT4 using the following threshold values: P value of 0.05, fold-change of 2 and gene rank in the top 10% among all differentially expressed genes, and Oncomine then listed all the data sets ordered by P value; for each published data set, the values were linked to the graphical representations of the original microarray data set. Each sample value was log 2 transformed. Heatmap figure was generated in OriginPro 2015. P values were calculated using Student’s t -test. Transwell invasion assay Matrigel was used to coat 24-well transwell inserts with 8-μm pores (Corning). An aliquot of 4 × 10 4 cells (diluted in 200 μl of DMEM medium containing 0.2% BSA) was seeded on top of the Matrigel in the upper side of the insert; the bottom side was filled with culture medium containing 10% foetal bovine serum as the chemo-attractant. After incubation for 48 or 72 h, non-invading cells were removed with a cotton swab, and the remaining cells were fixed, stained with crystal violet and photographed using an IX51 microscope. Dual luciferase assay Cells were seeded in 24-well plates at 60% confluency, then co-transfected with 500 ng of the Snail promoter reporter plasmid, 500 ng of expression plasmid and 25 ng of Renilla luciferase pRL-TK as an internal control. After 24 h incubation, the luciferase activities of the reporters were measured using the Dual Luciferase Reporter Assay System (Promega) according to the manufacturer’s protocol. Cell-cycle analysis Cells were seeded at 2 × 10 5 cells per well in a 6-well plate and incubated overnight. Cells then were transfected with 2 μg AF6-encoding plasmids and further incubated for 48 h. At analysis, cells were trypsinized, washed with PBS and fixed overnight at 4 °C with 1 ml per well 70% ethanol, followed by centrifugation at 2,000 g for 5 min, incubation with 100 μg ml −1 RNase (Sigma) and staining with 50 μg ml −1 propidium iodide (Sigma) for 15 min in the dark. The DNA content was analysed in a Cell Lab Quanta SC flow cytometer (Beckman Coulter, USA). MTT proliferation assay Cells (3,500 per well) were seeded in 96-well plates in triplicate, and incubated for indicated time intervals. MTT solution (20 μl at 5 mg ml −1 ; Sigma) then was added into each well and plates were incubated for 3 h at 37 °C. The supernatant was aspirated and the crystals were dissolved by the addition of 100 μl of DMSO. The absorbance was measured at 570 nm in a SpectraMax 190 microplate reader (Molecular Devices, USA). IHC analysis and mass spectrometry TMA chips containing pancreatic tumours and matched adjacent tissues were purchased from the Biobank Center of National Engineering Center for Biochip. Briefly, the IHC staining was performed using TMA sections that were deparaffinized in xylene, rehydrated with graded ethanol, washed in Tris-buffered saline and processed using a streptavidin–biotin–peroxidase complex method. Antigen retrieval was performed in sodium citrate buffer (pH 6.0). After quenching of endogenous peroxidase activity and blocking of nonspecific binding, sections were incubated with primary antibody at 4 °C overnight. Slides then were incubated with an appropriate dilution of the corresponding secondary antibody for 1 h at room temperature. After further washing with Tris-buffered saline, sections were incubated with StrepABComplex/horseradish peroxidase (Dako, Inc., USA) for 30 min at room temperature. Chromogenic immunolocalization was conducted using 0.05% 3,3′-diaminobenzidine (Dako). All sections were counterstained with haematoxylin. Other cores containing PC served as positive controls for gene expression; normal serum was used in the place of primary antibody as a negative control. The IHC evaluation of protein expression intensity in normal adjacent tissues and paired PC tissues was performed independently by two pathologists from the Department of Pathology, Zhongshan Hospital (Fudan University). The pathologists were blinded to the patient’s clinical features; in cases of disagreement, a consensus was reached by joint review. The staining intensity was scored as described previously [47] : 0, no positive cells detectable; 1, very few positive cells (<5%) showing weak light-brown staining; 2, a few positive cells (<10%) showing weak to medium brown staining; 3, a few positive cells (<10%) showing medium to dark brown staining; 4, large number of positive cells (>10%) showing medium to dark brown staining; 5, large number of positive cells (>20%) exhibiting medium to dark brown staining. When evaluating the expression of proteins in normal tissues and paired cancer tissues, ‘high’ means that the score of cancer tissues is higher than the score of the paired normal tissues; in converse, ‘low’ means that the score of cancer tissues is lower than the score of the paired normal tissues. When evaluating the intratumor expression of AF6 and Snail, we defined a score of 0–2 as low and 3–5 as high, respectively. Mass spectrometry was performed as previously described [48] ; all the candidates derived from the MS analysis are summarized in Supplementary Table 5 . Immunofluorescence imaging Cells were grown on coverslips or in chamber slides, fixed with 4% paraformaldehyde and incubated overnight with antibodies. Proteins were visualized by incubation with Alexa Fluor-conjugated secondary antibodies (Invitrogen), and the coverslips or slides were mounted with mounting medium containing DAPI (Prolong Gold Antifade Reagent, Life Technologies). Fluorescence was monitored by confocal laser microscopy (Carl Zeiss). Chromosomal IP The ChIP assay was performed using the EZ-ChIP Kit (Millipore) according to the manufacturer’s instructions. Immune reagents consisted of a rabbit monoclonal antibody against FOXE1 and a negative control (isotype) rabbit immunoglobulin-G (Cell Signaling Technology). Purified immunoprecipitated DNA was used for quantitative reverse transcription–PCR (RT–PCR). Primers for ChIP-PCR are shown in Supplementary Table 4 . Orthotopic xenograft transplantation Four-week-old female nude mice (BALB/c, nu/nu ) were purchased from the Shanghai Experimental Animal Center (Shanghai, China) and maintained in pathogen-free conditions. All animals were used in accordance with the guidelines of the Institutional Animal Care and Use Committee of the Institute of Nutritional Sciences. Orthotopic xenograft transplantation was performed as previously described [49] . Briefly, mice were anesthetized by intraperitoneal injection of ketamine (100 mg kg −1 ) and xylazine (20 mg kg −1 ). A median laparotomy was conducted, then in vitro -grown PC cells (1 × 10 6 cells per animal, re-suspended in 100 μl serum-free DMEM medium containing 30% (v/v) Matrigel) were slowly injected into the pancreas. Specifically, cells were injected into the tail of the pancreas and allowed to pass into the head region of the organ; to prevent leakage the needle was withdrawn slowly from the pancreas after injection. Sixty days after cancer cell injection, mice were killed and their tumour xenografts, livers, lungs and spleens were harvested for further evaluation. The livers, lungs and spleens were fixed with formalin, dehydrated, embedded in paraffin and sectioned. To examine metastasis, the resulting sections were subjected to haematoxylin and eosin staining and evaluated by light microscopy for the presence of micro-metastases. Notably, liver metastasis was evaluated using transverse sections of each liver; the sections were examined by light microscopy by two independent pathologists blinded to sample identities; in cases of disagreement, a consensus was reached by joint review. The numbers of micro-metastases were counted by randomly selected four fields from randomly selected three tissue sections of each liver, and the calculated mean value was defined as ‘average liver metastases’. Statistical analysis Error bars in figures represent s.d., as indicated in figure legends. Unpaired two-tailed Student’s t -tests were used to assess statistical significance in the cell and mouse tumorigenesis experiments. Survival curves were calculated by the Kaplan–Meier method, with comparisons performed using the log-rank test. A χ 2 -test was performed to analyse the correlation between AF6 or Snail expression and clinical pathological features in PC samples. P values were calculated with the GraphPad Prism 5 software (San Diego, CA, USA); P values of <0.05 were considered statistically significant. How to cite this article: Xu, Y. et al. Loss of polarity protein AF6 promotes pancreatic cancer metastasis by inducing Snail expression. Nat. Commun. 6:7184 doi: 10.1038/ncomms8184 (2015).